Homeostatic neurogenesis in the adult hippocampus does not involve amplification of Ascl1highintermediate progenitors Neural stem/progenitor cells generate neurons in the adult hippocampus. Neural stem cells produce transient intermediate progenitors (type-2 cells), which generate neuroblasts (type-3 cells) that exit the cell cycle, and differentiate into neurons. The precise dynamics of neuron production from the neural stem cells remains controversial. Here we lineage trace Notch-dependent neural stem cells in the dentate gyrus and show that over 7–21 days, the progeny of the neural stem cells progress through an Ascl1 high intermediate stage (type-2a) to neuroblasts. However, contrary to predictions, this Ascl1 high population is not an amplifying intermediate, but it differentiates into mitotic Tbr2 + early neuroblasts, which in turn expand the lineage. After 100 days, the majority of the neural stem cell progeny are neuroblasts or postmitotic neurons. Hence, the neural stem cells require many weeks to generate differentiated neurons. On the basis of this temporal delay in differentiation and population expansion, we propose that the neural stem cell and early neuroblast divisions drive dentate gyrus neurogenesis and not the amplification of type-2a intermediate progenitors as was previously thought. Neural stem/progenitor cells (NSCs) self-renew and generate newborn neurons in the adult subventricular zone lining the lateral ventricles and the subgranular zone (SGZ) of the hippocampal dentate gyrus (DG) [1] , [2] . Radial and horizontal SGZ NSCs (type-1 cells) produce type-2 intermediate progenitors (IPs) that maintain Sox2 expression and increase levels of the proneural factor Ascl1 [2] , [3] , [4] , [5] , [6] , [7] , [8] . Late IPs (type-2b and type-3 cells) express Dcx and Prox1, and these early neuroblasts leave the cell cycle to mature into granule neurons [2] , [3] , [5] , [9] . Although much is known about neurogenesis in the adult DG [2] , [3] , [5] , the process of forming new granule cells from NSCs in vivo is not clear. This is due to a lack of genetic tools specific for DG NSCs that allow lineage tracing in vivo and detailed analysis of the neurogenic process in adults. Transgenic mice expressing 4-hydroxy-tamoxifen (TAM)-inducible Cre-recombinase (CreER) enable temporospatial analysis of gene function and cell fate. The promoters of Nestin , GLAST , GFAP , TLX and Sox2 have all been used to drive CreER in neural progenitor cells, but they do not restrict expression to NSCs of the adult DG and may also target IPs [10] , [11] , [12] , [13] , [14] , [15] , [16] , [17] , [18] . This has resulted in discrepancies about the identity of stem and progenitor populations, and particularly about the nature of amplifying intermediates within the lineage. Lineage tracing of Nestin -expressing progenitors has shown that neurogenesis in the adult DG is a dynamic process initiated by multipotent NSCs [11] , [12] . The current view of DG neurogenesis is that somatic stem cells in the brain are quiescent, although this is now being challenged [4] , [6] . S-phase labeling paradigms indicated that some NSCs are mitotically active during homeostasis and have a cell cycle time of less than 24 h [4] , [12] . On the basis of the asymmetric cell division model, NSCs divide to self-renew and generate a rapidly dividing, but committed type-2 IP daughter cell [19] , [20] . The type-2 pool is divided into type-2a and type-2b cells, based on their rounded morphology and the expression of the neuroblast protein doublecortin (Dcx) by type-2b cells [20] . Detailed analysis of cell cycle markers support that some type-1, type-2 and type-3 cells are in the cell cycle and suggested that Dcx − type-2a progenitor cells are the most mitotically active transient amplifying population in the adult DG [20] . However, the timing of neurogenesis from active NSCs has been difficult to analyze, as viral labeling and thymidine analog incorporation are not restricted to NSCs and transgenic lineage tracing has been hampered by a lack of cell-type specificity. Hence, the prevailing model is that adult DG lineage amplification occurs through expansion of type-2a cells and limited cell division by stem cells and neuroblasts [2] , [20] . Notch signaling is a key mediator of NSC maintenance, suppressing the expression of proneural genes including Ascl1 , and supporting the progenitor cell survival [21] , [22] , [23] . Deletion of Notch1 or RBP-J from DG NSCs results in a loss of stem cells and neurogenesis [4] , [24] , [25] , [26] . Canonical Notch signaling distinguishes self-renewing multipotent NSCs in the adult DG from IPs and neuronal precursors, and Notch reporter alleles allow purification of NSCs from the adult DG [4] , [26] , [27] , [28] . Regulatory elements of the Hes5 gene restrict expression to NSCs in the DG [4] . We demonstrated earlier that in the DG SGZ, Hes5 ∷ GFP is expressed by NSCs and one of the earliest markers in the adult granule cell lineage [4] . Here we have generated Hes5 ∷ CreER T2 mice and lineage-traced adult DG NSCs with active Notch-signaling by conditional genetic labeling to address the population dynamics within the hippocampus. We reveal that although some DG NSCs are actively proliferating [4] , their generation of differentiated neurons is a protracted process taking many days and weeks. NSCs rapidly generate IPs (type-2a), which express elevated levels of the proneural gene Ascl1. In contrast to previous findings, we observed that these do not expand in number, but rather produce mitotic neuroblasts (Dcx + ). These immature neuroblasts (type-2b) express Tbr2 and expand to increase the progenitor pool before they exit the cell cycle (as late type-3 cells) and finally differentiate into neurons. Furthermore, newborn neurons appear in clusters implying regionalized expansion and common ancestry within the SGZ. Our lineage analysis suggests that early IP expansion and asymmetric cell division may not be exclusively linked to differentiation during homeostatic DG neurogenesis. Rather, DG neurogenesis relies on active stem cell division and the proliferation and expansion of immature Tbr2 + neuroblasts. Hes5 ∷ CreER T2 expression is restricted to NSCs in the adult DG In the adult DG SGZ, canonical Notch signaling through Hes5 is active in NSCs [4] . We generated Hes5 ∷ CreER T2 mice to lineage trace the hippocampal NSCs, placing a CreER T2 cDNA under the control of the regulatory elements of the mouse Hes5 gene (Methods and Supplementary Fig. S1 ). In a proof of principle, TAM treatment of Hes5 ∷ CreER T2 mice in utero resulted in recombination of a Cre-reporter allele ( Rosa26-CAG ∷ EGFP ; Supplementary Fig. S1 ) and labeling of cells and their progeny in the embryonic brain, some of which contribute to the postnatal hippocampus ( Supplementary Figs S2 and S3 ). Embryonic NSCs labeled at E14.5 continued to generate neurons in the adult DG ( Supplementary Fig. S3 ). We have previously demonstrated morphologically and functionally distinct NSCs subpopulations in the adult DG that display Hes5 ( Hes5 ∷ GFP ) expression [4] . Hes5 ∷ CreER T2 expression overlapped with Hes5 ∷ GFP in the adult DG ( Fig. 1a ). A total of 93.8±0.5% of the Hes5 ∷ GFP + cells expressed Hes5 ∷ CreER T2 , and 82.5±5.8% of the Hes5 ∷ CreER T2 + cells expressed Hes5 ∷ GFP ( Fig. 1b ). Hes5 ∷ CreER T2 was expressed by both the radial ( Fig. 1c , arrows) and the horizontal ( Fig. 1c , arrowhead) NSC subpopulations in the DG [4] . To demonstrate conditional induction of Cre-activity, we induced recombination of the Rosa26R locus in adult Hes5 ∷ CreER T2 Hes5 ∷ GFP transgenic mice by TAM administration ( Supplementary Fig. S1 ) [15] . β-Gal expression from the recombined Rosa26R locus was restricted to Hes5 ∷ GFP + cells ( Fig. 1d ). Thus, Hes5 ∷ CreER T2 is active in both radial and horizontal adult DG NSCs, enabling lineage tracing. 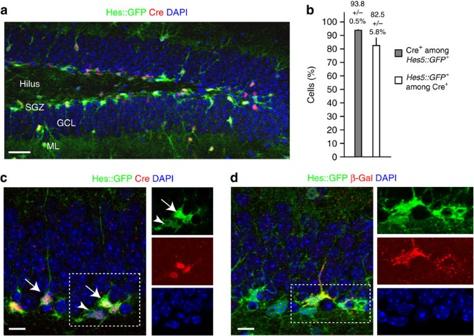Figure 1:Hes5∷CreERT2expression overlaps withHes5∷GFPin DG NSCs. (a) In adultHes5∷CreERT2Hes5∷GFPdouble-transgenic mice,Hes5∷GFP+cells in the SGZ express Cre-recombinase. (b) Quantification ofHes5∷GFP+and Cre co-expression. (c) Both radial (arrows) and horizontal (arrowhead)Hes5∷GFP+NSCs expressHes5∷CreERT2. (d) Cre activity is induced to lineage trace both radial and horizontalHes5∷GFP+NSCs, using the Rosa26R reporter allele (β-Gal). β-Gal, β-Galactosidase; GCL, granule cell layer; ML, molecular layer; SGZ, subgranular zone. Error bars are s.d. Scale bars in (a) equals 100 μm, in (c) and (d) equals20 μm. Figure 1: Hes5 ∷ CreER T2 expression overlaps with Hes5 ∷ GFP in DG NSCs. ( a ) In adult Hes5 ∷ CreER T2 Hes5 ∷ GFP double-transgenic mice, Hes5 ∷ GFP + cells in the SGZ express Cre-recombinase. ( b ) Quantification of Hes5 ∷ GFP + and Cre co-expression. ( c ) Both radial (arrows) and horizontal (arrowhead) Hes5 ∷ GFP + NSCs express Hes5 ∷ CreER T2 . ( d ) Cre activity is induced to lineage trace both radial and horizontal Hes5 ∷ GFP + NSCs, using the Rosa26R reporter allele (β-Gal). β-Gal, β-Galactosidase; GCL, granule cell layer; ML, molecular layer; SGZ, subgranular zone. Error bars are s.d. Scale bars in ( a ) equals 100 μm, in ( c ) and ( d ) equals20 μm. Full size image Hes5 + NSCs generate IPs in the SGZ To lineage trace the Hes5 + cells in the DG, we followed the Hes5 ∷ CreER T2 -mediated recombination of the Rosa26-CAG ∷ EGFP allele (hereafter referred to as rGFP + for recombined reporter-derived GFP) after TAM administration ( Fig. 2a and Supplementary Fig. S1 ). After 5 days of TAM-induction, most rGFP + cells expressed NSC/progenitor markers, including Sox2, BLBP and GFAP, and retained Cre expression, indicating that they had not commenced differentiation ( Fig. 2a,b and not shown). Hes5 ∷ CreER T2 was expressed by mitotically active (proliferating nuclear antigen; PCNA + ), as well as quiescent NSCs (PCNA − ; Fig. 2c,d ). Thus, we traced the fate of both the DG NSC populations. 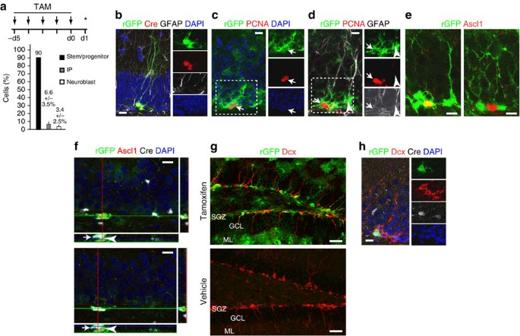Figure 2:Hes5∷CreERT2-expressing cells include mitotically active and quiescent NSCs and generate IPs. (a) TAM induction regime once per day for 5 consecutive days before the mice were killed (*) one day (d1) after the end of induction. Quantification of labeled cells on d1, the majority are still NSCs, and the first Ascl1+IPs appear. (b) The majority of the labeled cells at d1 still show Cre-expression, have NSC morphology, and expressed GFAP. (c,d) TAM-induced Cre-activity and recombination of theRosa26-CAG∷EGFPreporter allele (rGFP) in PCNA+NSCs (arrow;c). The labeled radial NSCs (arrowhead) are mitotically inactive (PCNA−), whereas some horizontal NSCs express PCNA (arrow;d). (e) Labeled rGFP+Ascl1+IPs appear on d1 and are in close proximity to rGFP+NSCs. Ascl1+cells that are not labeled (rGFP−) are in close proximity to NSCs and were likely generated before the TAM induction. (f) rGFP+Ascl1+IPs (arrowhead) do not express Cre, but are close to Cre+NSCs (arrow). (g) Most rGFP+cells at d1 are progenitors and few rGFP+Dcx+neuroblasts are present.Hes5∷CreERT2Rosa26-CAG∷EGFPanimals mock induced with vehicle only do not have rGFP+cells. (h) Clusters of Dcx+neuroblasts are in close proximity to Cre+rGFP+NSCs, suggesting a lineage relationship. GCL, granule cell layer; ML, molecular layer; SGZ, subgranular zone; TAM, tamoxifen. Error bars are s.d. Scale bars equals 20 μm, and in (g), equals 100 μm. Figure 2: Hes5 ∷ CreER T2 -expressing cells include mitotically active and quiescent NSCs and generate IPs. ( a ) TAM induction regime once per day for 5 consecutive days before the mice were killed (*) one day (d1) after the end of induction. Quantification of labeled cells on d1, the majority are still NSCs, and the first Ascl1 + IPs appear. ( b ) The majority of the labeled cells at d1 still show Cre-expression, have NSC morphology, and expressed GFAP. ( c , d ) TAM-induced Cre-activity and recombination of the Rosa26-CAG ∷ EGFP reporter allele (rGFP) in PCNA + NSCs (arrow; c ). The labeled radial NSCs (arrowhead) are mitotically inactive (PCNA − ), whereas some horizontal NSCs express PCNA (arrow; d ). ( e ) Labeled rGFP + Ascl1 + IPs appear on d1 and are in close proximity to rGFP + NSCs. Ascl1 + cells that are not labeled (rGFP − ) are in close proximity to NSCs and were likely generated before the TAM induction. ( f ) rGFP + Ascl1 + IPs (arrowhead) do not express Cre, but are close to Cre + NSCs (arrow). ( g ) Most rGFP + cells at d1 are progenitors and few rGFP + Dcx + neuroblasts are present. Hes5 ∷ CreER T2 Rosa26-CAG ∷ EGFP animals mock induced with vehicle only do not have rGFP + cells. ( h ) Clusters of Dcx + neuroblasts are in close proximity to Cre + rGFP + NSCs, suggesting a lineage relationship. GCL, granule cell layer; ML, molecular layer; SGZ, subgranular zone; TAM, tamoxifen. Error bars are s.d. Scale bars equals 20 μm, and in ( g ), equals 100 μm. Full size image Hes5 ∷ CreER T2 was not expressed by Ascl1 high type-2a IPs. After 6 days (5 days TAM+1 day chase; d1), a few rGFP + cells expressed Ascl1, and these did not express Cre-recombinase, implying that they were the differentiating progeny of Hes5 + NSCs ( Fig. 2a,e and f ). rGFP + Ascl1 high IPs were always singular but in close proximity to rGFP + NSCs ( Fig. 2e ). The later appearance of rGFP + Ascl1 high cells and their proximity to rGFP + NSCs indicated a lineage relationship between the two cell types. At this early point after induction, clusters of rGFP + Cre + NSCs were also located next to the rGFP − Dcx + neuroblasts ( Fig. 2g,h ). rGFP + Dcx + neuroblasts were rare at this point ( Fig. 2a,g and h ). Thus, Hes5 ∷ CreER T2 mediates the recombination in and labeling of DG NSCs that generate Ascl1 high type-2a IPs following a short chase. Hes5 + cells are neurogenic NSCs Generation of neurons from neural progenitors in the adult DG has been proposed to take 2–4 weeks, but timing has been hampered by the experimental approaches used [6] , [14] , [19] , [29] . We analyzed the Hes5 ∷ CreER T2 mice seven days (d7) and 3 weeks after TAM induction (d21; Fig. 3a ). The proportion of NSCs in the rGFP + population was reduced at both d7 (67.5%; Fig. 3a ) and d21 (51.7%), compared with d1 (compare Figs 2a and 3a,b ). However, the proportion of rGFP + cells that expressed the type-2a marker Ascl1 was similar at d1 (6.6±3.5%), d7 (7.0±2.4%) and d21 (3.5±1.3%), conducive with these being a transient population and indicative that IPs are generated continually from rGFP + NSCs. The low but constant number of rGFP + Ascl1 high cells over time suggested that this population does not accumulate. 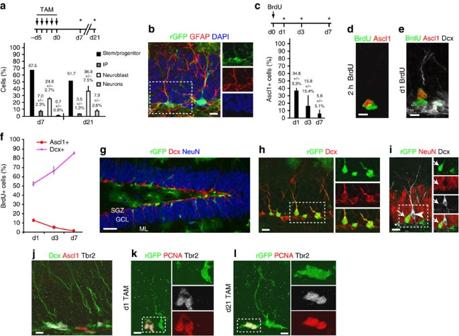Figure 3:Hes5∷CreERT2-labeled NSCs generate neuroblasts after 21 days. (a) TAM induction regime once per day for 5 consecutive days before the mice were killed (*) at 7 days (d7) or 21 days (d21) after the end of induction. Quantification of labeled cells on d7 and d21. At d7, the majority are still NSCs, whereas the first rGFP+NeuN+neurons start to appear at d21. (b) The majority of the labeled (rGFP+) cells at d21 still have NSC morphologies and expressed NSC markers, including GFAP. (c) BrdU induction regime. BrdU was administered once at day 0 (d0) and the mice were killed (*) 1 day (d1), 3 days (d3), or 7 days (d7) later. Quantification of Ascl1+cells labeled with BrdU on d1, d3 and d7. The proportion of BrdU-labeled Ascl1+cells decreased over time. (d) Some Ascl1+cells incorporated BrdU 2 h after induction. (e) At d1 after BrdU application, clusters of BrdU-labeled cells appear, which included a single Ascl1+cell and Dcx+neuroblasts. (f) Graphical representation of the fractions of Ascl1+and Dcx cells among the BrdU-incorporating cell populations. The proportion of the BrdU-labeled cells that were Ascl1+type-2a IPs decreased over time, whereas Dcx+neuroblasts increased. (g) rGFP+cells remain in the SGZ and are in close proximity to Dcx+neuroblasts. NeuN labels mature neurons in the DG granule cell layer. (h) rGFP+Dcx+neuroblasts are prominent in the SGZ by d21. (i) A proportion of the rGFP+cells are postmitotic differentiated neurons (arrow). A small population of Dcx+neuroblast remains unlabeled (arrowhead). (j) Tbr2+Dcx+early neuroblasts were clustered in close proximity to Ascl1+IPs. (k) Tbr2+cells were proliferating (PCNA+) in the adult SGZ, but rGFP+Tbr2+cells were rare at d1 after TAM induction. (l) At d21 after TAM induction, recombined rGFP+Tbr2+were present in the SGZ and proliferating (PCNA+). GCL, granule cell layer; ML, molecular layer; SGZ, subgranular zone; TAM, tamoxifen. Error bars are s.d. Scale bars equals 20 μm, and in (g), equals 100 μm. Figure 3: Hes5 ∷ CreER T2 -labeled NSCs generate neuroblasts after 21 days. ( a ) TAM induction regime once per day for 5 consecutive days before the mice were killed (*) at 7 days (d7) or 21 days (d21) after the end of induction. Quantification of labeled cells on d7 and d21. At d7, the majority are still NSCs, whereas the first rGFP + NeuN + neurons start to appear at d21. ( b ) The majority of the labeled (rGFP + ) cells at d21 still have NSC morphologies and expressed NSC markers, including GFAP. ( c ) BrdU induction regime. BrdU was administered once at day 0 (d0) and the mice were killed (*) 1 day (d1), 3 days (d3), or 7 days (d7) later. Quantification of Ascl1 + cells labeled with BrdU on d1, d3 and d7. The proportion of BrdU-labeled Ascl1 + cells decreased over time. ( d ) Some Ascl1 + cells incorporated BrdU 2 h after induction. ( e ) At d1 after BrdU application, clusters of BrdU-labeled cells appear, which included a single Ascl1 + cell and Dcx + neuroblasts. ( f ) Graphical representation of the fractions of Ascl1 + and Dcx cells among the BrdU-incorporating cell populations. The proportion of the BrdU-labeled cells that were Ascl1 + type-2a IPs decreased over time, whereas Dcx + neuroblasts increased. ( g ) rGFP + cells remain in the SGZ and are in close proximity to Dcx + neuroblasts. NeuN labels mature neurons in the DG granule cell layer. ( h ) rGFP + Dcx + neuroblasts are prominent in the SGZ by d21. ( i ) A proportion of the rGFP + cells are postmitotic differentiated neurons (arrow). A small population of Dcx + neuroblast remains unlabeled (arrowhead). ( j ) Tbr2 + Dcx + early neuroblasts were clustered in close proximity to Ascl1 + IPs. ( k ) Tbr2 + cells were proliferating (PCNA + ) in the adult SGZ, but rGFP + Tbr2 + cells were rare at d1 after TAM induction. ( l ) At d21 after TAM induction, recombined rGFP + Tbr2 + were present in the SGZ and proliferating (PCNA + ). GCL, granule cell layer; ML, molecular layer; SGZ, subgranular zone; TAM, tamoxifen. Error bars are s.d. Scale bars equals 20 μm, and in ( g ), equals 100 μm. Full size image Previous bromodesoxyuridine (BrdU) incorporation data implied that type-2a cells are highly proliferative and responsible for the expansion of the neurogenic lineage by symmetric division [20] . Therefore, we performed BrdU pulse-chase experiments ( Fig. 3c ) and compared the results with those from our Hes5 ∷ CreER T2 lineage-tracing experiments. Ascl1 high IPs incorporated BrdU ( Fig. 3d,e ); however, these were a small fraction of the total BrdU + cells (d1; Fig. 3f and Supplementary Table S1a ). The proportion of BrdU + Ascl1 high IPs decreased over time, whereas the proportion of BrdU + Dcx + neuroblasts (includes type-2b and type-3 cells) increased ( Fig. 3f and Supplementary Table S1a ). Thus, together, BrdU labeling and genetic lineage tracing indicated that Ascl1 high cells pass though S-phase of the cell cycle, but do not accumulate as a population or accumulate by symmetric cell division. In contrast to Ascl1 high type-2a IPs, the number of rGFP + Dcx + neuroblast increased dramatically between d1 (3.4±2.5%) and d21 (36.9±7.5%; compare Figs 2a and 3a,g,h ). At d7, when the proportion of NSCs in the rGFP + population was reducing, Dcx + neuroblasts were accumulating, indicative of a delayed expansion of intermediates (24.8±2.7%; Supplementary Table S1b-d ). Hence, NSCs had started to generate type-2a IPs at d1, but not many neuroblasts (including type-2b and type-3 cells). The bulk of the Dcx + neuroblasts appeared within the next 6 days and peaked over the next 21 days, whereas Ascl1 high IPs remained constant. Before d7, we had not found rGFP + NeuN + neurons, and at d7, they were still a minor population (0.7±0.9%; Figs 2a and 3a ). Even 21 days after induction, the number of Hes5 -derived labeled neurons was low (7.9±2.6%; Fig. 3a,g and i ). Therefore, Hes5 + -labeled NSC progeny had progressed to neuroblast and the first newborn neurons in 3 weeks, but they showed a delay in differentiation, spending a considerable time as neuroblasts. To elucidate the stage at which lineage amplification occurs in the DG, we examined the Tbr2 + cells. Tbr2 labels type-2b cells in the adult SGZ and it overlaps with Dcx in early neuroblasts ( Fig. 3j ) [30] , [31] . Tbr2 was not expressed by Ascl1 high type-2a IPs, although Ascl1 high and Tbr2 + cells where found in close proximity, suggesting a lineage relationship between the two populations ( Fig. 3j ). Tbr2 + Dcx + type-2b cells were mitotically active (PCNA + ) and often formed large clusters ( Fig. 3j,k ). Hes5 -derived rGFP + Tbr2 + cells were rare at d1 after Cre-induction and appeared in clusters later ( Fig. 3k,l ), which was in sharp contrast to Ascl1 high type-2a cells. These results imply that amplification in the adult DG neurogenic lineage occurs at the type-2b/early neuroblast stage rather than at the previously thought type-2a stage. Newborn neurons accumulate over 100 days and NSCs remain in the DG NSCs of the DG generate granule neurons throughout life. By d21 after Cre-induction, the majority of the rGFP + cells were NSCs and only a minor fraction expressed the neuronal differentiation marker NeuN. We extended the lineage trace period to 100 days after TAM treatment ( Fig. 4a ). By d100, rGFP + Dcx + neuroblasts were present in and around the SGZ ( Fig. 4b ), and rGFP + NeuN + newborn neurons were more numerous in the granule cell layer ( Fig. 4c–e ). The number of rGFP + cells increased over the tracing periods due to accumulation and amplification of the progeny of the NSCs ( Fig. 4f ). At d100, NeuN + were the largest single population of the rGFP + cells (44.0±1.8%; Fig. 4g,h ). rGFP + NSCs remained in the DG at d100 and their proportion (29.2%) of the rGFP + cells reduced as a consequence of the accumulation of neuroblasts and postmitotic neurons ( Fig. 4g ). However, quantification revealed that the number of NSCs remained relatively constant over the 100 days ( Fig. 4h ). Similarly, the proportion of the rGFP + Dcx + neuroblasts reduced between d21 and d100 also, as a result of accumulating neurons, but their actual numbers continued to increase up to d100 ( Fig. 4h ). The continued presence of rGFP + Ascl1 high and rGFP + Tbr2 + IPs, and rGFP + Dcx + neuroblasts in the DG after 100 days of lineage tracing indicated continual replenishment of these populations from the NSC pools ( Fig. 4a,g and h ). 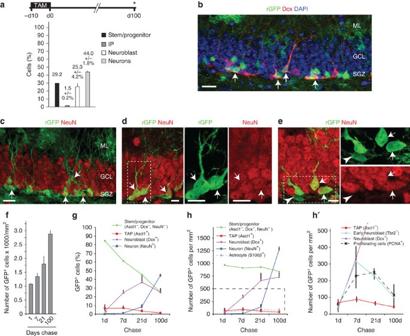Figure 4:Hes5∷CreERT2NSCs generate granule neurons. (a) TAM induction regime once per day for 10 consecutive days before the mice were killed (*) 100 days (d100) after the end of induction. Quantification of labeled cells on d100, NeuN+neurons are the largest single rGFP+population. (b) 100 days after induction, new neuroblasts (Dcx+; arrows) are still being generated, indicating labeling of NSCs. (c,d) rGFP+NeuN+neurons are found in clusters, and migrate into the granule cell layer (arrows). (e) rGFP+NeuN−cells remain in the SGZ 100d after TAM induction (arrowhead) in close proximity to newly generated rGFP+NeuN+neurons (arrows). (f) Consistent with having labeled NSCs, rGFP+cells accumulate over the 100d of lineage tracing. (g) Lineage and population development ofHes5∷CreERT2-derived rGFP+cells over time. (h) Graphical representation of the development, production and maintenance of the individualHes5∷CreERT2-derived cell types in the DG lineage (absolute numbers). (h′) Representation of the area indicated in (h) showing the development of proliferating cells (PCNA) in the DG lineage relative to Ascl1 (type-2a)-, Tbr2 (type-2b)- and Dcx (neuroblast)-expressing cells (absolute numbers). GCL, granule cell layer; ML, molecular layer; SGZ, subgranular zone; TAM, tamoxifen. Error bars are s.d. Scale bars in (b) and (c) equals 100 μm, in (d) and (e) equals 10 μm. Figure 4: Hes5 ∷ CreER T2 NSCs generate granule neurons. ( a ) TAM induction regime once per day for 10 consecutive days before the mice were killed (*) 100 days (d100) after the end of induction. Quantification of labeled cells on d100, NeuN + neurons are the largest single rGFP + population. ( b ) 100 days after induction, new neuroblasts (Dcx + ; arrows) are still being generated, indicating labeling of NSCs. ( c , d ) rGFP + NeuN + neurons are found in clusters, and migrate into the granule cell layer (arrows). ( e ) rGFP + NeuN − cells remain in the SGZ 100d after TAM induction (arrowhead) in close proximity to newly generated rGFP + NeuN + neurons (arrows). ( f ) Consistent with having labeled NSCs, rGFP + cells accumulate over the 100d of lineage tracing. ( g ) Lineage and population development of Hes5 ∷ CreER T2 -derived rGFP + cells over time. ( h ) Graphical representation of the development, production and maintenance of the individual Hes5 ∷ CreER T2 -derived cell types in the DG lineage (absolute numbers). ( h′ ) Representation of the area indicated in ( h ) showing the development of proliferating cells (PCNA) in the DG lineage relative to Ascl1 (type-2a)-, Tbr2 (type-2b)- and Dcx (neuroblast)-expressing cells (absolute numbers). GCL, granule cell layer; ML, molecular layer; SGZ, subgranular zone; TAM, tamoxifen. Error bars are s.d. Scale bars in ( b ) and ( c ) equals 100 μm, in ( d ) and ( e ) equals 10 μm. Full size image However, the type-2a (Ascl1 high ) IP and type-2b (Tbr2 + Dcx + ) early neuroblast populations showed a striking difference in dynamics during the lineage tracing ( Fig. 4h′ ). Although the number of Ascl1 high cells remained relatively constant over the 100 days, Tbr2 + cells peaked between days 7 and 21 ( Fig. 4h′ ). The initial increase in Tbr2 + cells paralleled Dcx + cells and mitotic progenitors (PCNA + ) because of strong overlap in expression at early stages [30] . The number of cells in Tbr2 + population mirrored that of the PCNA + cells over the entire 100 days, whereas the Ascl1 high population did not ( Fig. 4h′ ). Many newborn rGFP + NeuN + neurons in the DG were found in clusters, close to the rGFP + progenitors ( Fig. 4e ). Lineage tracing of Hes5 ∷ CreER T2 + cells following a single TAM injection resulted in sparse labeling of NSCs in the SGZ ( Supplementary Fig. S4a-c ). These clones contained an average of 1.14±0.35 cells. None of the rGFP + cells at day 2 after a single TAM injection were Ascl1 + or Dcx + , although rGFP + NSCs were associated with rGFP − neuroblasts. Over time (21 days), the rGFP + cells generated clusters that contained an average of 2.68±1.06 cells ( Supplementary Fig. S4d-f and Supplementary Table S2 ). A total of 19.5% of the clones (8 out of 41 clones from three animals) contained a single Ascl1 high type-2a cell, making an average of 0.2±0.4 Ascl1 high cells per clone ( Supplementary Table S2a,b ). Not a single clone contained more than one Ascl1 high cell. A total of 53.7% of the clones (22 out of 41 clones from three animals) at day 21 contained Dcx + cells, and five clones contained more than one Dcx + cell. On average, the individual clones contained 0.68±0.76 Dcx + cells after 21 days ( Supplementary Table S2 ). Many clones at day 21 contained either single or multiple cells but did not contain Ascl1 + or Dcx + cells ( Supplementary Table S2c ). Clones that included Ascl1 + cells usually contained multiple cells including stem cells and Dcx + neuroblasts. A total of 22 of the 41 clones analyzed contained Dcx + neuroblasts clones, and 2 consisted exclusively of Dcx + cells ( Supplementary Table S2b,c ). This supports the idea that Hes5 + cells are NSCs in clonal neurogenic units. The culmination of data propose an alternative dynamics in the populations generated in the adult DG, with a transition from NSCs to IPs, neuroblasts and neurons, and expansion at the Tbr2 + Dcx + early neuroblast and not the Ascl1 high type-2a IP stage ( Fig. 5 ). 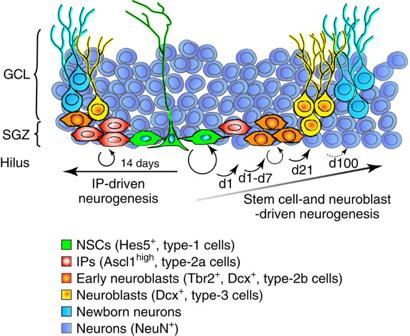Figure 5: Lineage progression from Hes5∷CreERT2NSCs in the adult DG. Scheme of IP and stem cell-driven homeostatic DG neurogenesis. Type-1Hes5+NSCs can be quiescent or active. In the current IP driven model, NSCs generate type-2a Ascl1highIPs through asymmetric cell division. Type-2a IPs undergo symmetric self-replicating progenitor divisions before generating a pool of committed progenitors (type-2b cells also referred to as D1 cells53). These early neuroblasts (Tbr2+) undergo a limited number of divisions and give rise to post-mitotic neuroblasts and newborn granule cells. In the stem cell and early neuroblast-driven model, active NSCs divide multiple times, but will generate type-2a Ascl1highIPs that produce mitotic Tbr2+early neuroblasts (type-2b cells) without amplification of the pool. The type-2b early neuroblasts divide to increase and expand the precursor pool before generating post-mitotic neuroblasts and newborn neurons. The average time taken for these process deduced from the lineage-tracing experiments is shown in days. GCL, granule cell layer, SGZ, subgranular zone. Figure 5: Lineage progression from Hes5 ∷ CreER T2 NSCs in the adult DG. Scheme of IP and stem cell-driven homeostatic DG neurogenesis. Type-1 Hes5 + NSCs can be quiescent or active. In the current IP driven model, NSCs generate type-2a Ascl1 high IPs through asymmetric cell division. Type-2a IPs undergo symmetric self-replicating progenitor divisions before generating a pool of committed progenitors (type-2b cells also referred to as D1 cells [53] ). These early neuroblasts (Tbr2 + ) undergo a limited number of divisions and give rise to post-mitotic neuroblasts and newborn granule cells. In the stem cell and early neuroblast-driven model, active NSCs divide multiple times, but will generate type-2a Ascl1 high IPs that produce mitotic Tbr2 + early neuroblasts (type-2b cells) without amplification of the pool. The type-2b early neuroblasts divide to increase and expand the precursor pool before generating post-mitotic neuroblasts and newborn neurons. The average time taken for these process deduced from the lineage-tracing experiments is shown in days. GCL, granule cell layer, SGZ, subgranular zone. Full size image Newborn neurons in the adult are important for brain function [24] , [32] , [33] , [34] , [35] , [36] . Neurogenesis is regulated by physiological stimuli and by pathologies [37] , [38] , [39] , [40] , [41] . Understanding the dynamics of the neurogenic process is important to understand the mechanisms active in brain homeostasis and disease. Neurogenesis in the DG proceeds from NSCs through transient IPs to committed neuroblasts and differentiated granule neurons. Amplification in the lineage is thought to occur through multiple symmetric divisions of IPs, primarily at the type-2a stage [5] , [42] , [43] . To shed light on the neurogenic process, several transgenic mouse lines have been used to lineage trace NSCs in a controlled manner [10] , [13] , [14] , [15] , [16] , [17] , [18] , [44] , [45] , [46] , [47] . However, the expression of most transgenes is not restricted in the SGZ to NSCs, resulting in labeling of more differentiated cell types [5] , [20] . This has complicated analysis of the timing of DG neurogenesis, and a clear understanding of the critical steps in the generation of new neurons is still lacking. Canonical Notch signaling and its downstream target Hes5 are restricted in the SGZ of the DG to NSCs [4] , [48] . Therefore, we used inducible CreER technology and lineage-traced Hes5 + Notch-signaling cells in the adult DG. As expected, Hes5 ∷ CreER T2 was expressed by NSCs, but not by IPs, neuroblasts and differentiated neurons. Hes5 + NSCs maintain their progenitor identity and contribute to homeostatic hippocampal neurogenesis over a prolonged period in vivo ( Fig. 4g ). This enabled a detailed examination of neurogenesis to understand the dynamics of the process and analyze the intermediate stages of neuron production in the DG. We traced ∼ 1,000 Hes5 + NSCs per mm 2 in the DG SGZ and this number remained constant over 100 days. Previously, we showed that 15% of the Hes5 + SGZ NSCs are active, do not express markers of IPs (Ascl1 high or Dcx), but have a cell cycle time of <24 h [4] . Therefore, Hes5 + SGZ NSCs contribute neurons and remain in the DG SGZ, indicating that they must self-renew. This confirms our previous findings that Hes5 + SGZ NSCs remain even in the brains of old mice and indicates that the reduction in neurogenesis seen with age is due, at least in part, to quiescence or dormancy of NSCs [4] . These results are in contrast to reports showing a dramatic and rapid reduction in Nestin + progenitors in the DG of aging mice, NSC depletion and an increase in astrocyte differentiation at the expense of neurogenesis [12] . We did not observe increases in Hes5 ∷ CreER T2 -derived polymorphic astrocytes (S100β + ) over time, confirming results from clonal analysis of SGZ NSCs [11] . We also did not observe Hes5 + NSC-derived oligodendrocytes; hence, in accordance with other reports, adult DG NSCs are mainly neurogenic and do not contribute majorly to gliogenesis in vivo [6] , [11] , [14] , [17] , [47] , [49] . We predicted that NSCs would generate Ascl1 high type-2a cells. However, on the basis of our previous data [4] , we also predicted that expansion of the DG granule lineage occurs primarily at the NSC and Dcx + neuroblast levels and not through classic IPs (type-2a cells). Indeed, Ascl1 high cells were the first progeny of the Hes5 + cells in the SGZ. However, in contrast to being a transient amplifying pool of cells, their number remained constant and did not increase during the lineage-tracing experiments. In addition, Ascl1 high cells were singular and did not occur in clusters even in the lineage-tracing experiments, which would have been expected of an amplifying cell type. Confirming previous reports, we found that these type-2a Ascl1 high cells are in the cell cycle and incorporate BrdU. However, to explain their constant numbers in the lineage tracing and the rapid loss of BrdU-labeled Ascl1 high cells, one or both daughters must downregulate Ascl1 expression upon cell division. This is likely as a result of differentiation to early neuroblasts. Alternatively, Ascl1 high type-2a cells may be eliminated by apoptosis [50] . Lineage tracing of Ascl1 + cells has confirmed their progenitor status, mostly as IPs. However, some SGZ NSCs express Ascl1 and the Ascl1 ∷ CreER knock-in locus can trace long-term neurogenic NSCs [51] . This is in complete agreement with our findings and the current understanding of oscillatory Notch signaling. High levels of Ascl1 expression are associated with IP status [49] and neuronal commitment, whereas the oscillatory expression of the canonical Notch targets, including the Hes genes in NSCs, results in an unstable refractory expression of their repressed targets including Ascl1 [52] . Therefore, NSCs could express Ascl1 at low, oscillatory levels. Labeled neuroblasts (defined by the expression of Dcx) were not present at the beginning, but appeared early in our lineage-tracing experiments. We analyzed the neuroblast population further, based on the Tbr2 and Dcx expression. Our findings confirm previous data, which indicated a substantial overlap in Tbr2 and Dcx expression in early neuroblasts [30] . Therefore, we subdivided the neuroblasts into early neuroblasts (Tbr2 + Dcx + ; type-2b) and type-3 neuroblasts (Tbr2 − Dcx + ; D1 cells). Early neuroblasts (type-2b cells) were mitotically active, found in clusters, and their numbers peaked during the lineage-tracing analysis as would be expected for a transient amplifying population. In addition, the lineage profile of Tbr2 + cells reflected that of the mitotic cells (PCNA + ). The almost constant relationship between the Trb2 and PCNA over the entire lineage-tracing experiment lends strong support for Tbr2 + Dcx + being a major amplifying population in the adult SGZ [30] , [31] . It is interesting to note that type-2b cells do not express the progenitor protein Nestin, which is often associated with multipotency [5] . These results are very significant, as they indicate that neuronally committed cells may be a major population through which the number of newborn neurons is regulated. This is also in agreement with retroviral-labeling studies, showing limited clonal potential of rapidly dividing cells [53] . On the basis of our previous data showing that ∼ 15% of the Hes5 + cells are proliferative, we predicted that under homeostatic conditions, more than 150 genetically labeled progeny of the 1000 labeled NSC (per mm 2 ) would have been generated per day [4] . After 6 days, only 122 Ascl1 high and Tbr2 + (includes the early Dcx + cells) cells were present in the DG. Cell death of IPs and neuroblasts has been shown in vivo ; however, retrospective quantification of apoptotic cells is difficult because of their rapid removal. Our data support that apoptotic selection likely occurs at the IP stages [50] . We cannot exclude that Ascl1 high IPs in the DG undergo non-productive cell divisions, where one or both daughters die. Indeed, BrdU labeling revealed that Ascl1 high cells divide, but indicated that this BrdU-labeled population rapidly declines with no evidence for expansion. Hence, BrdU pulse-chase data also supports the conclusion that expansion of type-2a IPs is not the driving force for DG neurogenesis under normal conditions. In summary, mitotic Hes5 + NSCs in the DG provide some early lineage expansion and generate progeny, initiating neurogenic differentiation. Neuronal production from Hes5 + NSCs in the DG passes through Ascl1 high and Tbr2 + Dcx + intermediates, and requires more than 21 days under homeostatic conditions ( Fig. 5 ). Our results indicate that Hes5 + NSCs are a driving force for neurogenesis, but also suggest that under normal conditions and in contrast to previous models, although Ascl1 high type-2a IPs remain in the cell cycle (incorporate BrdU), the population does not amplify the lineage. Amplification in the lineage takes place at the level of committed early neuroblasts (type-2b cells). This is consistent with recent data showing IP expansion of neurogenesis in response to pathophysiological stimuli [54] . Similar to our previous findings that distinct NSC population respond to specific physiological stimuli [4] , the mode of increasing neuronal numbers may change under circumstances where rapid production of many neurons is required [54] . However, under normal conditions, the pool of NSCs requires 100 days before the number of newborn neurons exceeds their number. Therefore, after the initiation of neurogenesis, cells remain at the immature Dcx + NeuN − neuron stage for weeks or months, allowing them to adapt to physiological or pathophysiological stimuli that may affect their maturation and differentiation. Further analysis will be required to establish which cues regulate the various stages of neurogenesis beyond NSC expansion and survival of newly formed neurons. It is likely that in addition to the recruitment of the IP expansion, increasing IP survival may be affected by different phathophysiological input. We propose that the prolonged period in an immature state and the ability to recruit IPs to expand may provide a store of immature neurons poised to integrate into circuits or to replace lost neurons. Cloning and generation of Hes5 ∷ CreER T2 transgenic mice To generate the Hes5 ∷ CreER T2 construct, a Sal I linker fragment was inserted into the unique Bam HI restriction site of pBS-Hes5 [27] . TAM-inducible Cre-recombinase, CreER T2 , was amplified by PCR from pGS-CreER T2 , with Sal I restriction sites added to both ends of the open-reading frame before cloning into the Sal I site of the pBS-Hes5 construct to generate pBS-Hes5 ∷ CreER T2 . pBS-Hes5 ∷ CreER T2 was linearized by Eco RI and Psp XI, and the 5.1-kb fragment containing the entire Hes5 ∷ CreER T2 construct purified over agarose gel and injected into the male pronucleus of fertilized oocytes. Transgenic founder mice were identified by PCR and crossed to Rosa26-CAG ∷ EGFP . Nine founder mice were identified and all passed the transgene on to their offspring. Four of the nine lines that were established on a C57/Bl6 genetic background showed comparable CreER T2 expression in the expected Hes5 patterns [27] , [55] , [56] , [57] . We have focused on the analysis of line 2, although comparable results were obtained with the other three lines. Animals and husbandry Hes5 ∷ GFP and Rosa26R mice have been described elsewhere [27] , [58] . Rosa26-CAG ∷ EGFP mice were generated by introducing an eGFP reporter gene into a modified Rosa26 locus using recombinase-mediated cassette exchange [59] to allow Cre-dependent enhanced green fluorescent protein expression from the chicken β-actin promoter. Young, adult mice between 8 and 10 weeks of age were used for the experiments. Mice were maintained on a 12-h day/night cycle with adequate food and water under specified pathogen free conditions and according to the Max-Planck Institutional and German Federal regulations, and under license numbers 35/9185.81/G-09/19 (Ethical Commission Freiburg, Germany). TAM and BrdU administration Stock solutions of TAM (Sigma) were prepared at a concentration of 20 mg ml −1 in corn oil (Sigma). Adult mice were injected i.p. with TAM once per day for 5 or 10 consecutive days (as indicated in the experiments) at a dose of 2 mg per day. For low-dose TAM induction, adult mice were injected i.p. with a single dose of 2-mg TAM. Embryonic induction at E14.5 was with a single i.p. injection of TAM (3 mg) to the pregnant mice. The animals were killed 3 days or 9 weeks after induction. Mice that were induced during adulthood were killed at 1, 2, 7, 21 or 100 days after the last injection, and the brains prepared for immunohistochemistry as described below. BrdU (Sigma) was administered to the adult animals via a single i.p. injection (50 mg per kg body weight). The animals were killed 2 h, 1, 3 or 7 days after the administration, and the brains prepared for immunohistochemistry as described below. Tissue preparation and immunhistochemistry For histology, mice were deeply anesthetized by injection of a ketamine/xylazine/unitrazepam solution (150 mg, 7.5 and 0.6 mg per kg body weight, respectively) and perfused with ice-cold 0.9% saline solution, followed by ice-cold 4% paraformaldehyde solution in 0.1 M phosphate buffer (PB). Brains were post-fixed with 4% paraformaldehyde overnight, washed in PB, cryoprotected in a 30% sucrose solution in 0.1 M PB for 48 h, embedded and frozen in OCT (TissueTEK). Free-floating coronal sections (30 μm) were collected in multi-well dishes (Corning) and stored at −20 °C in antifreeze solution until use. For immunostaining, sections were incubated overnight at 4 °C, with the primary antibody diluted in blocking solution of 2% normal donkey serum (Jackson ImmunoResearch), 0.5% Triton X-100 in phosphate-buffered saline. Sections were washed three times in phosphate-buffered saline and incubated at room temperature for 1 h with the corresponding secondary antibodies in blocking solution. When necessary, sections were washed and incubated for 1 h at room temperature in streptavidin–FITC (Jackson ImmunoResearch; 1:500) and counter-stained with DAPI (1 μg ml −1 ). For PCNA detection, antigen was recovered at 80 °C for 20 min in sodium citrate solution (10 mM, pH7.4). For BrdU detection, sections were treated with 2 M HCl at 37 °C for 30 min before primary antibody incubation. HCL-treated sections where then equilibrated in borate buffer (0.1 M, pH8.5) for 10 min. The antibodies used are listed in Supplementary Tables S3 and S4 . Stained sections were mounted on Superfrost glass slides (Thermo Scientic), embedded in mounting medium containing diazabicyclo-octane (DABCO; Sigma) as an anti-fading agent and visualized using a Zeiss LSM510 confocal microscope. Quantification and data analysis Randomly selected, stained cells were analyzed with fixed photomultiplier settings on a Zeiss LSM510 confocal microscope (Zeiss). The total number of recombined (rGFP + ) cells in the SGZ was estimated using a ×40 magnification objective. The area of the granule cell layer was measured using ImageJ software and used to estimate the number of labeled cells per mm 2 . For clonal analysis after low-dose TAM induction, cells within a clone were defined as rGFP + cells within 100 μm of a central rGFP + cell. Data are presented as average percentages of co-labeled cells. In all graphs, error bars are s.d. Tables of the values are shown in Supplementary Tables S1 and S2 . How to cite this article: Lugert, S. et al . Homeostatic neurogenesis in the adult hippocampus does not involve amplification of Ascl1 high intermediate progenitors. Nat. Commun. 3:670 doi: 10.1038/ncomms1670 (2012).